Late glacial initiation of Holocene eastern Mediterranean sapropel formation Recurrent deposition of organic-rich sediment layers (sapropels) in the eastern Mediterranean Sea is caused by complex interactions between climatic and biogeochemical processes. Disentangling these influences is therefore important for Mediterranean palaeo-studies in particular, and for understanding ocean feedback processes in general. Crucially, sapropels are diagnostic of anoxic deep-water phases, which have been attributed to deep-water stagnation, enhanced biological production or both. Here we use an ocean-biogeochemical model to test the effects of commonly proposed climatic and biogeochemical causes for sapropel S1. Our results indicate that deep-water anoxia requires a long prelude of deep-water stagnation, with no particularly strong eutrophication. The model-derived time frame agrees with foraminiferal δ 13 C records that imply cessation of deep-water renewal from at least Heinrich event 1 to the early Holocene. The simulated low particulate organic carbon burial flux agrees with pre-sapropel reconstructions. Our results offer a mechanistic explanation of glacial–interglacial influence on sapropel formation. Various climatic events have been proposed as causes for stagnating deep-water formation and/or enhanced biological production leading to sapropel formation in the eastern Mediterranean Sea (EMS) [1] , [2] , [3] , [4] , [5] . The timing of most quaternary sapropel events, including the most recent deposited S1 (10.2–6.4 kyr ago) [6] , [7] , is correlated with minima in the orbital precession cycle [8] , [9] , [10] . This orbital configuration induces a northward shift of the African monsoon into the southern catchment of the EMS, and enhances river run-off and nutrient input [8] , [11] , [12] . The Nabtian Pluvial Period (NP; 14–8 kyr ago) [11] is the last wet period across much of the southern EMS catchment, and is characterized by an intense humid phase with strongly enhanced Nile run-off after 12 kyr ago [11] , [12] . The enhanced Nile run-off may have capped the EMS with freshwater, causing a weakening or shutdown of deep-water formation and ventilation [1] , [2] , [3] , [4] , [5] , [8] . Other freshwater sources were also proposed to have diminished deep-water formation such as enhanced precipitation [13] , [14] , inflow of meltwater from regional or remote continental glaciers [15] , [16] and the EMS reconnection with the Black Sea [17] , [18] , [19] . Enhanced continental run-off would have washed more land-derived nutrients into the EMS, boosting particulate organic carbon (POC) production and increasing oxygen consumption by respiration of sinking POC [20] . The time required for full S1 deep-water oxygen depletion was often inferred to take less than 2,000 years [2] , [7] , [21] , [22] , [23] . This timing is consistent with strongly enhanced Nile run-off induced by the NP. Alternatively, it has been shown by a simple palaeohydraulic model that the climatic changes associated with the last deglaciation resulted in ∼ 6 kyr of stagnation before S1 deposition [2] . Thus, this concept places the onset of the deep-water stagnation into the Heinrich event 1 (H1, 18–15.5 kyr ago) [24] . The last glacial to early Holocene transition was characterized by ∼ 3 °C global warming [25] , and melting of the Laurentide and Fennoscandian ice sheets, which caused ∼ 100 m of sea-level rise and freshening of the North Atlantic [26] . The rising sea level (most rapid during two periods—Meltwater pulse (MWP) 1A, ∼ 14 kyr ago [26] , [27] , [28] ; MWP-1B, ∼ 11 kyr ago [26] , [27] or rather ∼ 9.5 kyr ago [28] ) invigorated the water exchange at the Strait of Gibraltar, and this in turn enhanced the freshening of Mediterranean Sea surface water relative to that of the North Atlantic Ocean [29] , [30] , [31] , [32] , [33] . Changes in Mediterranean deep-water properties lagged those at the surface due to a slower response time, leading to strengthened vertical stratification and reduced deep-water ventilation [2] , [32] . A similar concept was suggested for the formation of the last organic-rich layer (ORL1; 14.5–8.2 kyr ago) deposited in the Alboran Sea [5] , [31] , [34] . The ending of ORL1 deposition corresponds to cold and dry conditions, which are also recorded as an interruption of S1 deposition above 2,000 m water depth [6] , [7] , [35] . The onset of S1 deposition throughout the EMS appears to have been nearly synchronous, irrespective of depth [6] , [7] , [36] , except for the Adriatic Sea where S1 deposition started later [35] . Deep sediment cores from the EMS also suggest that intermittent ventilation events during S1 deposition rarely reached the deep EMS, and that deep water was persistently devoid of oxygen [6] , [23] , [36] . In contrast, the continual occurrence of benthic foraminifera [23] , [37] and low-sediment POC content [36] in waters <2,000 m deep imply dysoxic to only intermittently anoxic conditions during S1, which indicates that dense-water formation in the northern region, at least occasionally, persisted [36] . It was suggested that at these shallower locations, in areas of rapid POC posting to depth, anoxia only developed in ‘blankets’ draped over the sea floor [37] . This dynamic concept could explain rapid reoxygenation of the sea floor even in areas remote from deep-water formation, and also rationalize regional differences in POC flux and oxygen conditions indicated by benthic repopulation events and changes in redox state during S1 and other sapropels [35] , [37] , [38] , [39] , [40] . Rapid posting of POC from the euphotic zone to the sea floor in a stratified ocean was explained by diatom production within a deep chlorophyll maximum (DCM) [41] . Evidence for changed ecological niche occupation in the pelagic system has been seen in earlier sapropels, and also in S1 of the easternmost Mediterranean Sea [42] , [43] . Several attempts have been made to trace the processes leading to sapropel deposition using numerical models. Physical ocean-only studies showed that with increasing strength of the freshwater forcing the strength of the deep-water stagnation is increased, and that changes in the source of freshwater modulate this effect [44] , [45] , [46] . A reduced strength of deep-water formation was simulated by imposing the last glacial–interglacial sea-level rise [32] , or a gradual freshening of the Atlantic water inflow [46] . Questions on the interplay between physical circulation and deep-water oxygen consumption have been addressed by two ocean-biogeochemical modelling studies [21] , [22] . Both studies concluded that stagnating deep-water circulation, combined with a large external nutrient input, is a prerequisite for S1 formation. However, in both of these studies, the static stagnating ocean circulation set-ups chosen did not permit conclusions on the stability of deep-water stagnation over time, which is the most crucial process to assess the time evolution and duration of the deep-water oxygen deficiency. The time required to develop full deep-water anoxia was significantly reduced by simulating a rapid downward transport of POC that led to a combined development of anoxia below the ventilation–stagnation interface (VSI) and the bottom water [22] . This finding, with an anoxic bottom-water layer forming beneath parts of the deep-water column that still contain oxygen, might explain the occurrence of anoxic blankets [37] . However, under the static ocean circulation in the one-dimensional model [22] , frequent reventilation of the anoxic blankets are not simulated. Here we make the first attempt to identify the mechanisms leading to S1 formation using a regional three-dimensional prognostic ocean circulation model coupled to a biogeochemical model including a sediment module. Through a series of idealized model experiments and their rigorous evaluation with sediment data, we gain a conceptual understanding of the external (climatic) and internal (circulation and biological production) mechanisms determining S1 formation. We find that with the observed low pre-sapropel POC burial flux, complete S1 deep-water oxygen depletion requires at least 5.5 kyr of persistent deep-water stagnation; this is confirmed by a new composite δ 13 C record of epibenthic deep-sea foraminifera, showing that the deep-water stagnation leading to S1 anoxia was emplaced during or near the end of H1. Baseline experiment The general circulation and biogeochemical patterns of the Baseline experiment resemble those of the present-day EMS, and the simulated upper-ocean climate agrees well with early Holocene proxy temperature reconstructions [47] . As in the present-day situation, the deep EMS ( Supplementary Fig. 1 ) is mainly ventilated ( Fig. 1a,b , Supplementary Fig. 2a ) and oxygenated by deep-water formation in the Adriatic Sea ( Supplementary Fig. 3a , Supplementary Fig. 4a,b and Supplementary Note 1 ). Along the deep-water flow path from the Ionian Sea to the Levantine Sea, continuous oxygen utilization is simulated, resulting in the lowest deep-water oxygen concentrations in the Levantine Sea ( Fig. 2a,b , Supplementary Fig. 5a,b ). 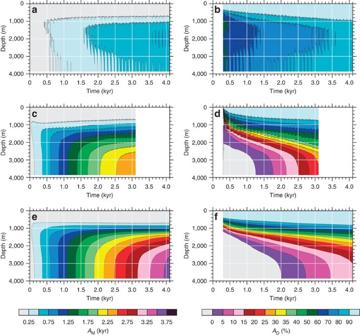Figure 1:ΑMandΑDaveraged over the Ionian Sea. Hovmöller diagrams ofΑM(left column) andΑD(right column) of the Baseline experiment (same for 3xNutri experiment) (a,b), Nile experiment (c,d), IniGlac experiment (same for IniGlac+3xNutri experiment) (e,f). The Ionian averaging area is marked inSupplementary Fig. 1. Results for the Levantine Sea are displayed inSupplementary Fig. 2. Similar to today, low riverine nutrient inputs ( Supplementary Table 1 ) combined with an anti-estuarine circulation pattern exporting nutrients from the EMS support only low levels of biological production, POC export production ( Fig. 3a,b ) and POC burial in the sediment ( Fig. 4a , Supplementary Fig. 6a and Supplementary Note 2 ). Figure 1: Α M and Α D averaged over the Ionian Sea. Hovmöller diagrams of Α M (left column) and Α D (right column) of the Baseline experiment (same for 3xNutri experiment) ( a , b ), Nile experiment ( c , d ), IniGlac experiment (same for IniGlac+3xNutri experiment) ( e , f ). The Ionian averaging area is marked in Supplementary Fig. 1 . Results for the Levantine Sea are displayed in Supplementary Fig. 2 . 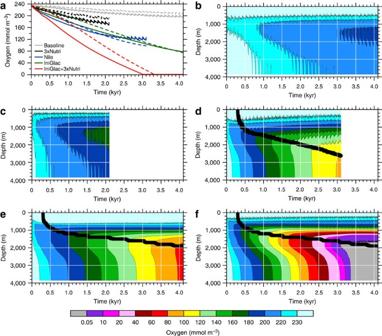Figure 2: Annual mean oxygen concentration averaged over the Ionian Sea. Time series of the oxygen concentration in 1,800 m (solid line) and 2,920 m (dashed line) (a). Hovmöller diagram of the oxygen concentration for the Baseline experiment (b), 3xNutri experiment (c), Nile experiment (d), IniGlac experiment (e) and IniGlac+3xNutri experiment (f). The thick black line indicates the depth of the VSI. The extent of the Ionian averaging area is marked inSupplementary Fig. 1. Results for the Levantine Sea are displayed inSupplementary Fig. 5. Full size image Figure 2: Annual mean oxygen concentration averaged over the Ionian Sea. Time series of the oxygen concentration in 1,800 m (solid line) and 2,920 m (dashed line) ( a ). Hovmöller diagram of the oxygen concentration for the Baseline experiment ( b ), 3xNutri experiment ( c ), Nile experiment ( d ), IniGlac experiment ( e ) and IniGlac+3xNutri experiment ( f ). The thick black line indicates the depth of the VSI. The extent of the Ionian averaging area is marked in Supplementary Fig. 1 . Results for the Levantine Sea are displayed in Supplementary Fig. 5 . 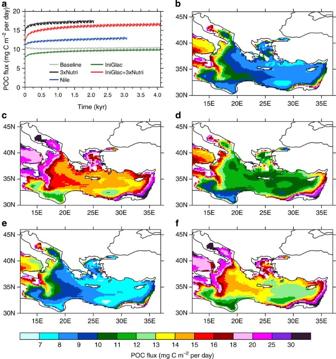Figure 3: Annual mean POC export production at the base of the euphotic zone. Time series of the POC export production (POC flux at 102 m depth) over the course of each experiment smoothed with a 20-year running mean (a). Map of POC export production for the Baseline experiment (b), 3xNutri experiment (c), Nile experiment (d), IniGlac experiment (e) and IniGlac+3xNutri experiment (f). Results (b–f) are averaged between the simulation years 2,001 and 2,100. Note the non-linear colour scale. Full size image Figure 3: Annual mean POC export production at the base of the euphotic zone. Time series of the POC export production (POC flux at 102 m depth) over the course of each experiment smoothed with a 20-year running mean ( a ). Map of POC export production for the Baseline experiment ( b ), 3xNutri experiment ( c ), Nile experiment ( d ), IniGlac experiment ( e ) and IniGlac+3xNutri experiment ( f ). Results ( b – f ) are averaged between the simulation years 2,001 and 2,100. Note the non-linear colour scale. 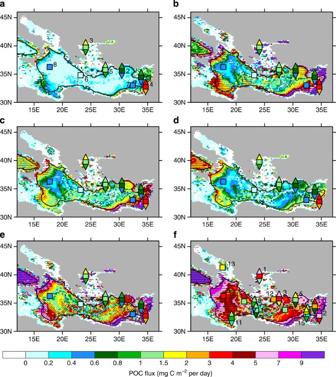Figure 4: Sediment POC burial flux. 100-year means of the POC burial flux of the Baseline experiment (years 4,001 to 4,100) (a), 3xNutri experiment (years 2,001 to 2,100) (b), Nile experiment (years 3,001 to 3,100) (c), IniGlac experiment (years 4,001 to 4,100) (d), IniGlac+3xNutri experiment (years 2, 801 to 2,900) (e) and IniGlac+3xNutri experiment (years 4,001 to 4,100) (f). Model results are overlain with POC burial fluxes inferred from sediment cores, where mean fluxes (squares) and maximum/minimum values (upward/downward pointing triangles) represent the pre-sapropel period between 10.5 and 11.5 kyr ago (a–e), and the sapropel period between 6.5 and 9.5 kyr ago (f), unless not otherwise given in the respective data source (seeSupplementary Note 2andSupplementary Fig. 6for details). The black line marks the 1,500 m contour line. Line- and point-shaded areas indicate where the model drift is <−0.05 and >0.05 mg C m−2per day over the last 500 years of simulation. Numbers represent sediment cores given inSupplementary Fig. 6. Full size image Figure 4: Sediment POC burial flux. 100-year means of the POC burial flux of the Baseline experiment (years 4,001 to 4,100) ( a ), 3xNutri experiment (years 2,001 to 2,100) ( b ), Nile experiment (years 3,001 to 3,100) ( c ), IniGlac experiment (years 4,001 to 4,100) ( d ), IniGlac+3xNutri experiment (years 2, 801 to 2,900) ( e ) and IniGlac+3xNutri experiment (years 4,001 to 4,100) ( f ). Model results are overlain with POC burial fluxes inferred from sediment cores, where mean fluxes (squares) and maximum/minimum values (upward/downward pointing triangles) represent the pre-sapropel period between 10.5 and 11.5 kyr ago ( a – e ), and the sapropel period between 6.5 and 9.5 kyr ago ( f ), unless not otherwise given in the respective data source (see Supplementary Note 2 and Supplementary Fig. 6 for details). The black line marks the 1,500 m contour line. Line- and point-shaded areas indicate where the model drift is <−0.05 and >0.05 mg C m −2 per day over the last 500 years of simulation. Numbers represent sediment cores given in Supplementary Fig. 6 . Full size image 3xNutri experiment With the eutrophication scenario (3xNutri), we test whether it is plausible that S1 formation was caused by increased biological production only, without changing the circulation (hypothesis 1, Table 1 ). The modelled enhanced POC export production ( Fig. 3a,c ) increases the deep-water respiratory oxygen consumption rate, but oxygen deficiency does not evolve in deep water ( Fig. 2a,c , Supplementary Fig. 5a,c ); this is because winter deep-water formation in the Adriatic Sea continues ( Supplementary Fig. 3a , Supplementary Fig. 4a,b ) so that oxygen utilization and deep-ventilation equilibrate at moderately high oxygen levels after ∼ 2 kyr of simulation ( Fig. 2a,c , Supplementary Fig. 5a,c ). The simulated deep-water oxygen content agrees with previous model results with well-ventilated but stronger POC production scenarios [21] , [22] . Depletion of the initial oxygen concentration to suboxic levels without changing the circulation requires an unrealistically high external nutrient input. Thus, the 3xNutri experiment implies that a stagnating deep-water circulation is a prerequisite for S1 formation. Table 1 Experimental design used to simulate the main hypotheses for S1 formation. Full size table Nile experiment With the Nile experiment (hypothesis 2, Table 1 ), we test whether S1 formation was caused during the intense wet phase of the NP. The simulation results show that enhanced Nile discharge increases the buoyancy of the upper ocean to a point where a stable vertical density stratification is established and deep ventilation is inhibited. Over time, continuous winter dense-water formation in the Adriatic Sea ( Supplementary Fig. 3b , Supplementary Fig. 4c,d ) and mixing erode the vertical density gradient, which progressively enhances the deep-water ventilation along the flow path from the Ionian ( Fig. 1c,d ) to the Levantine Sea ( Supplementary Fig. 2b ), and deepens the VSI (see Methods; Fig. 2d ), so that oxygenated upper-ocean water progressively penetrates into greater depths ( Fig. 2a,d , Supplementary Fig. 5a,d ). The simulated VSI shows that reventilation to a depth of 2,600 m is established after 3.1 kyr of simulation ( Fig. 2d ). In 2,660 m depth, oxygen concentrations are depleted at a maximum rate of 57 mmol m −3 kyr −1 in the Ionian Sea, which is reached after ∼ 0.6 kyr of simulation, when POC export production has equilibrated ( Fig. 3a ), and deep-water stagnation is still strong ( Fig. 1c,d ). The maximum deep-water oxygen consumption rate is nearly tripled compared with previously published model results [21] of a comparable circulation, POC export production, and terrestrial nutrient input scenario. Extrapolating the deep-water oxygen consumption rate, it takes at least 4 kyr of simulation until deep-water anoxia is established in the Nile experiment. The observed time span between the onset of the strongly enhanced Nile river run-off (12 kyr ago) and the onset of S1 deposition (10.2 kyr ago) is thus obviously too short for complete oxygen depletion in the deep water body from an initial well-oxygenated state. Furthermore, since deep-water ventilation is re-established after ∼ 3.1 kyr ( Fig. 2d ), S1 anoxia will not evolve in this experiment. Although the enhanced Nile river nutrient input raises POC export over the entire basin compared with the Baseline experiment ( Fig. 3a,d ), the upper-ocean increase in biological production in the Nile experiment is subdued. This muted response is caused by nutrient trapping in the deep stagnating water body so that the biological production supported by cross-pycnocline mixing of regenerated nutrients is low. The simulated POC burial flux is in the range of fluxes reconstructed from sediment cores over large areas in the EMS, but is too high in the Nile plume area ( Fig. 4c , Supplementary Fig. 6c ). IniGlac experiment With the IniGlac experiment (hypothesis 3, Table 1 ), we test whether the S1 deep-water stagnation was preconditioned by the climatic changes associated with the last deglaciation. We initialized the model with deep-water properties (cold and salty) resembling the H1 state, and impose the same boundary conditions as those in the Baseline experiment (see Methods). Since we impose the climatic difference between H1 and the early Holocene abruptly, the IniGlac experiment does not mimic the natural climate variability throughout the last deglaciation, but immediately develops a strong vertical density stratification ( Fig. 1e,f , Supplementary Figs 2c , 3c and 4e,f ). The VSI linearly deepens over time ( Fig. 2e ). The simulated POC burial flux agrees with reconstructions for the pre-sapropel period ( Fig. 4d , Supplementary Fig. 6d ). Although the POC export production of the IniGlac experiment is reduced compared with the Baseline experiment ( Fig. 3a,e ), the cold deep water limits POC remineralization in the sediment (see Methods); this results in slightly higher POC burial rates than in the Baseline experiment ( Fig. 4a,d ). The deep-water oxygen is continuously utilized within the deep stagnating EMS ( Fig. 2e , Supplementary Fig. 5e ). In 2,660 m depth, the maximum oxygen consumption rate is 42 mmol m −3 kyr −1 (reached after ∼ 1.6 kyr of simulation, when POC export production has equilibrated ( Fig. 3a ), and the deep-water isolation is still very strong ( Fig. 1e,f )), trending to anoxia after at least 5.5 kyr of simulation. IniGlac+3xNutri experiment With the IniGlac experiment (hypothesis 4, Table 1 ), we test whether stagnant conditions combined with basin-wide strongly enhanced biological production, is a plausible scenario to explain S1 formation. Under the strongly enhanced POC export production ( Fig. 3a,f ) and stagnating deep-water conditions ( Fig. 1e,f , Supplementary Fig. 2c , Supplementary Fig. 4e,f ), the experiment develops complete basin-wide deep-water anoxia ( Fig. 2a,f , Supplementary Fig. 5a,f ), at an oxygen consumption rate similar to that of a previous model study with a 40% higher POC export production and a stagnating deep-water circulation [21] . In the Levantine Sea, the onset of anoxia is synchronous basin-wide at depths below ∼ 1,800 m after 3.1 kyr ( Supplementary Fig. 5f ). In the Ionian Sea, a rapid downward expansion of the anoxic layer from ∼ 1,700 m depth within ∼ 3.1–3.4 kyr is simulated ( Fig. 2f ). Overall, the simulated onset of anoxia agrees with the synchronous onset (dating precision ±200 years) of anoxia below 1,800 m inferred from proxy records [7] , [36] , [48] . The simulated sediment POC burial flux during both the pre-sapropel period and S1 deposition ( Fig. 4e,f , Supplementary Fig. 6e,f and Supplementary Note 2 ) is generally too high to match the reconstructions. Although the simulated POC burial flux under anoxic conditions is drifting towards lower values in the Ionian Sea ( Fig. 4f ), it may suggest enhanced POC production during S1 deposition. However, changes in the oxic–anoxic interface depth can also strongly influence the POC burial flux. For example, if we simulate a mid-water oxic–anoxic interface in the IniGlac experiment that is too shallow, the POC flux reaching the sediment is also strongly increased. Once anoxia has developed at intermediate depths in the Ionian Sea, reduced POC remineralization increases the POC burial flux. In geochemical proxy records, this effect could erroneously be interpreted as enhanced production immediately before the onset of S1 deposition. In areas between 1,800 and 1,600 m water depth, where the VSI impinges on the sea floor, an anoxic bottom layer is simulated. On multi-decadal to centennial timescales, cold events lead to the formation of denser water masses ( Supplementary Note 1 , Supplementary Fig. 4e,f ), which in turn enhance intermittent ventilation close to the VSI, thus ventilating the simulated local anoxia on the sea floor. However, the oxygen content in this layer remains rather low, and thus after the cold event the now stagnant water reverts to anoxia in a relatively short time. This model result is consistent with observations of rapidly fluctuating conditions and the formation of anoxic ‘blankets’ draped over the sea floor at intermediate depths [37] . δ 13 C records as proxy for persistence of stagnation Initiation of persistent stagnation and ongoing remineralization of sinking POC (at the expense of dissolved oxygen) must be registered in the deep-water pool of dissolved inorganic carbon and its isotopic composition. We verify the onset time of the deep-water stagnation simulated in our model experiments with a compilation of existing benthic foraminiferal δ 13 C data from various sites and water depths of the EMS ( Fig. 5 ). Commonly, the ageing and decrease in oxygen concentration of a deep-water mass is accompanied by a decrease in the δ 13 C of epibenthic foraminiferal carbonate, which reflects 12 C release during remineralization of settling organic matter [49] . The δ 13 C data set contains only strictly epifaunal taxa to exclude any pore-water bias on the signature of the bottom-water mass [50] . In addition, surface-water δ 13 C changes at deep-water formation sites will be communicated to bathyal or abyssal environments via newly formed deep water. The corresponding δ 13 C record of the epipelagic planktonic foraminifer Globigerinoides ruber from areas of intermediate and deep-water formation in the northern Levantine Sea and southern Aegean Sea reveals minor variability during the late glacial period, but a significant drop of at least 0.5% at the time of sapropel S1 formation [51] , [52] ( Fig. 5 ). This δ 13 C decrease has been attributed to the input of isotopically light dissolved inorganic carbon in freshwater run-off during the early Holocene [53] , [54] , although changes in biological production, niche occupation and seasonality cannot be ruled out. 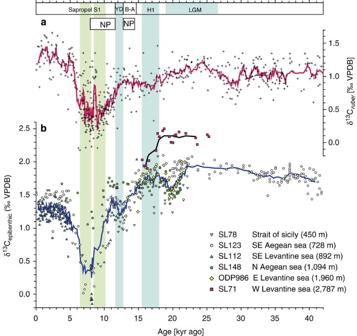Figure 5: Composition of benthic foraminiferal δ13C records from the EMS for the last 42 kyr. Compilation of epipelagic planktonic foraminiferal (Globigerinoides ruberwhite) δ13Cruberdata and seven-point running mean (red line) from areas of intermediate and deep-water formation in the Levantine Sea and South Aegean Sea51,52,69(a). Compilation of intermediate and deep-water epibenthic δ13Cepibenthicdata and seven-point running means (blue and black lines) from various regions and water depths of the EMS (b). δ13C data is fromPlanulina ariminensis,Cibicidoides pachydermus and C. kullenbergiin cores SL78 (new data), SL112, SL123 and SL148 (refs7,54), and ODP 986 (new data) (blue line), and fromMiliolinella subrotundain core SL71 (new data) (black line). Note thatM. subrotundaδ13C values are shifted to more positive values due to species-specific vital effects. Figure 5: Composition of benthic foraminiferal δ 13 C records from the EMS for the last 42 kyr. Compilation of epipelagic planktonic foraminiferal ( Globigerinoides ruber white) δ 13 C ruber data and seven-point running mean (red line) from areas of intermediate and deep-water formation in the Levantine Sea and South Aegean Sea [51] , [52] , [69] ( a ). Compilation of intermediate and deep-water epibenthic δ 13 C epibenthic data and seven-point running means (blue and black lines) from various regions and water depths of the EMS ( b ). δ 13 C data is from Planulina ariminensis , Cibicidoides pachydermus and C. kullenbergi in cores SL78 (new data), SL112, SL123 and SL148 (refs 7 , 54 ), and ODP 986 (new data) (blue line), and from Miliolinella subrotunda in core SL71 (new data) (black line). Note that M. subrotunda δ 13 C values are shifted to more positive values due to species-specific vital effects. Full size image The deep-sea epibenthic δ 13 C record is partly decoupled from the surface water signal and reveals the sequence of stagnation and reventilation events in the deep-water environment since the last glacial period ( Fig. 5 ). A first transient reduction in deep-water formation occurred as early as the last glacial maximum (LGM), ∼ 22–18 kyr ago. A more persistent phase of deep-water stagnation is evident near the end of H1 at ∼ 16 kyr ago. This signal is particularly strong in the only abyssal record available. The overall evolution of the epibenthic δ 13 C record confirms the results of the IniGlac model experiment and illustrates an early and sustained development of a stagnant deep-water mass at least ∼ 6 kyr before the onset of S1 formation. Short periods of deep-water renewal occurred during the Younger Dryas (YD; 12.8–11.6 kyr ago) [11] and a cold event centred on about 8.2 kyr ago ( Fig. 5 ). These events resulted in intermittently improved oxygenation of bathyal benthic ecosystems that led to their repopulation by benthic foraminifera around 8.2 kyr ago [35] . On the other hand, the persistently low δ 13 C values during these cold events imply only partial renewal and rather low deep-water oxygen concentrations. On the basis of a suite of idealized experiments with a regional three-dimensional prognostic ocean-biogeochemical model, we argue that the evolution of S1 deep-water anoxia required a long prelude of deep-water stagnation; the progressive deep-water oxygen depletion was caused by restricted deep-ventilation between H1 and S1, and required no permanently and strongly enhanced input of terrestrial nutrients, which is both confirmed by the sediment core data ( Figs 4 and 5 , Supplementary Fig. 6 ) and published data (see below). Our experiments also identify commonly proposed hypotheses as implausible scenarios for S1 formation: We show that enhanced biological production alone cannot overcome the effect of continuous deep-water ventilation (3xNutri experiment), implying that a stagnating deep-water body is a prerequisite for S1 formation. While massively increased Nile river freshwater and nutrient influx (Nile experiment) induces deep-water stagnation and enhances the production of POC, it cannot explain S1 formation, since the time span required for complete deep-water oxygen depletion exceeds the time span between the beginning of the intense wet phase of the NP and the onset of the anoxic period equivalent to S1 deposition. Even if we would underestimate the strength of the stagnation and biological production, the Nile hypothesis could still not explain S1 formation, since also the IniGlac+3xNutri experiment takes longer (3.4 kyr) to develop deep-water anoxia. In all experiments, the maximum oxygen consumption rate is significantly larger than previously shown under comparable ocean-biogeochemical model scenarios [21] , emphasizing that we present conservative low time estimates for the duration of the pre-sapropel stagnation. The long time span required to develop deep-water anoxia also excludes combinations of enhanced Nile river run-off with other latest Pleistocene to early Holocene climatic changes (for example, reconnection with the Black Sea) as cause for S1 formation, and suggests that deglaciation climatic effects must have essentially preconditioned the S1 deep-water stagnation. Although the IniGlac+3xNutri experiment perturbation pushes the EMS into basin-wide deep-water anoxia, the imposed nutrient influx is too high to be in accordance with the pre-sapropel POC burial flux. A lower POC production than simulated in the IniGlac+3xNutri experiment implies a longer time required for the development of deep-water anoxia, which again suggests that the S1 oxygen depletion was preconditioned earlier in real time during the last deglaciation. The trend of the maximum deep-water oxygen consumption in the oligotrophic IniGlac experiment suggests that at least 5.5 kyr of permanent and strong deep-water isolation are required for full deep-water oxygen consumption from an initial well-oxygenated state. A less strongly isolated deep-water mass would prolong the time required to develop deep-water anoxia (for example, the trend of the oxygen consumption at the end of the IniGlac experiments implies 6.5 kyr of stagnation required to develop deep-water anoxia). The required duration of the stagnation places its onset during or near the end of H1 (>15.7 kyr ago). As in the Nile experiment, the derived minimum time estimate for the required duration of the deep-water stagnation to develop S1 anoxia is estimated from the maximum trend of deep-water oxygen consumption. Hence, it is not primarily the modelled initiation of the deep-water stagnation, but the time required to develop deep-water anoxia, which gives rise to the climatic conditions during or near the end of H1 that essentially preconditioned the stagnant conditions cumulating in S1 anoxia. The so-derived duration of the deep-water stagnation between H1 and S1 is consistent with the timing and severity of deep-water isolation reflected in the composite δ 13 C record of epibenthic deep-sea foraminifera. During the last deglaciation, proxy records suggest that deep-water stagnation was only interrupted by one short period of incomplete deep-water renewal (thus deep-water oxygenation) during the YD cold event ( Fig. 5 ). Owing to the non-transient atmospheric forcing of our experiments, the YD climatic event was not accounted for in our experimental set-ups. Nonetheless, we performed sensitivity experiments to simulate the imprint of the YD climate on the mixing strength of the IniGlac experiment ( Supplementary Note 3 , Supplementary Fig. 7 and Supplementary Fig. 8 ). In accordance with the proxy records, we find enhanced partial reventilation at mid depths; however, the deep stagnating ocean remains almost unaffected by the simulated YD scenarios. The derived onset of deep-water stagnation from both the IniGlac experiment and δ 13 C proxy data are in line with the timing of the onset of deep-water stagnation derived from a simple palaeohydraulic model [2] , and with a weakening of WMDW formation at ∼ 16 kyr ago and subsequent collapse of WMDW formation ∼ 1.5 kyr later [34] . Hence, the deep circulation of the entire Mediterranean Sea was simultaneously affected by the climatic changes associated with the last deglaciation. The model data comparison of POC burial fluxes singles out the oligotrophic IniGlac experiment as the best scenario for the pre-sapropel state. Indeed, benthic foraminiferal successions and geochemical data across the glacial-Holocene transition indicate successively more oligotrophic conditions, except for the YD, and imply that enhanced organic matter fluxes are not a precondition for sapropel S1 formation [7] , [23] , [55] . The model data comparison of POC burial fluxes of the Nile experiment further shows that basin-wide raised nutrient levels may have slightly enhanced the pre-sapropel biological production, but that strongly increased nutrient influx from the Nile river overestimates the POC burial flux in the eastern Levantine Sea. Slightly higher biological production evenly distributed over the entire basin during the deglaciation was very likely achieved by cross-isopycnal mixing of highly nutrient-rich deep water. During the glacial, nutrients accumulated in the EMS by the same process as salinity, because the exchange rate across the Strait of Gibraltar was reduced by a factor of ∼ 2 due to the lower sea level [33] , [44] . The rising sea level during the deglaciation steadily increased nutrient export from the Mediterranean basin, and successively reduced the comparatively high deglacial POC flux to depth in the EMS. We initialized the IniGlac experiment with nutrient-poor conditions (see Methods), because no estimates of H1 nutrient concentrations are available for the EMS. Thus, the initial conditions of the biogeochemical model resemble an early Holocene state, while the physical ocean model resembles the H1 state. In all stagnation experiments (Nile, IniGlac and IniGlac+3xNutri experiments), the POC flux is initially reduced ( Fig. 3a ) because the rapidly established deep-water stagnation leads to a strong nutrient exhaustion of the upper ocean. Over time, the simulated biological production is enhanced since the progressive deepening of the VSI supports a continuously enhanced upward mixing of highly nutrient enriched deep water, which was trapped in the deep stagnating ocean. This effect would be enhanced if we would initialize the IniGlac experiments with the higher H1 nutrient content. However, since by far, the largest part of the biological production in a stagnating ocean is fuelled by external nutrient input, we expect that the model-derived time span required to develop deep-water anoxia would only shorten by a few hundred years. Enhanced oxygen consumption was possibly also supported by the development of productive DCMs, from where POC is rapidly exported to the deep ocean, as was shown in earlier model experiments for S1 (ref. 22 ). We also perform similar experiments and find that changes in the deep-water oxygen utilization rate are small ( Supplementary Figs 9–11 , Supplementary Note 4 ), and that the faster POC fallout leads to a stronger accumulation of POC in the sediment ( Supplementary Fig. 12 ). Besides, basin-wide changes in the pelagic ecosystem have only been found for the LGM and some earlier sapropels [41] , [42] , [43] so that enhanced POC production (via higher late glacial nutrient availability, see above) and transfer (from a DCM) would have accelerated the basin-wide oxygen consumption only during the well-ventilated LGM to H1, rather than during the entire prelude to S1. In our IniGlac+3xNutri experiment, we find the formation of a frequently reventilated anoxic bottom layer [37] in the depth range between (partially) oxygenated and anoxic water masses near the VSI. Differing from a previous one-dimensional model study on S1 formation [22] , an enhanced POC sinking speed does not lead to the formation of anoxia at the sea floor much longer before full deep-water anoxia evolves ( Supplementary Note 4 ). On the basis of the processes underlying the formation of local and frequently ventilated bottom-water anoxia in the IniGlac+3xNutri experiment, we suspect that such features would also develop in the oligotrophic IniGlac experiment, as soon as deep-water anoxia is established. With respect to the onset of anoxia in the IniGlac experiment, time-transgressive trends in stratification and oxygen consumption imply anoxia only at water depths below 2,000 m after 5.5 kyr, whereas the observed basin-wide oxic/anoxic interface was probably situated at a depth of 1,800 m (ref. 36 ). Also the duration of S1 would be underestimated by the IniGlac experiment, since the trend of the VSI suggests reventilation in the upper 2,600–3,000 m after ∼ 7 to ∼ 9 kyr of simulation. Possibly these discrepancies partly result from the time-slice set-up of the IniGlac experiment, and the mixing parameterization in the model. We initialized the model with cold and salty H1 water, and imposed the early Holocene Atlantic hydrography, sea level and atmosphere. Consequently, the IniGlac experiment immediately establishes a strong vertical density gradient, and the simulated VSI linearly deepens over time dependent on the properties of the simulated deep Adriatic outflow and the parameterized strength of the cross-isopycnal mixing. Although both of these processes can change the duration and strength of the simulated deep-water isolation, they cannot significantly enhance the presented maximum deep-water oxygen consumption rate, since the rate is derived from the simulation at the time of very strong deep-water isolation. Thus, uncertainties in the simulated persistence of the deep-water stagnation do not compromise the validity of our conclusion that a long prelude of deep-water stagnation is required for S1 formation. Our time-slice set-up does not elucidate the roles that the succession and interplay of climatic and biogeochemical fluctuations, or sea-level changes throughout the last deglaciation play for the time variability of both the VSI position and deep-water oxygen consumption. But the conceptual understanding drawn from our set of experiments and proxy data allows us to summarize the main mechanisms leading to S1 deep-water anoxia. For the time between the LGM and H1, enhanced POC fallout [23] from highly productive DCMs [42] possibly slightly reduced the deep-water oxygen content in a similar manner as simulated in the 3xNutri experiment. Around the termination of H1, the progressing deep-water oxygen consumption cumulating in S1 deep-water anoxia evolved due to warming and freshening ( Supplementary Fig. 13a , Supplementary Note 5 ; through sea-level rise and freshened Atlantic water inflow most pronounced during MWP-1A [26] , [27] , [28] , [32] , enhanced northern borderland river run-off [16] , precipitation and warming during the B-A [14] , and the onset of enhanced Nile run-off after 14 kyr ago [11] ), which caused the density contrast between the deep-water emplaced during the late glacial and an increasingly buoyant surface water during the deglaciation (IniGlac experiment). After VSI deepening and partial reventilation at mid depths during the YD ( Fig. 5 , Supplementary Note 3 ), surface warming and freshening (due to both the rising sea level and the freshening of the Atlantic water inflow most pronounced during MWP-1B [26] , [27] , [28] , [32] ), coincident with or followed by other moisture sources during the latest Pleistocene to the mid Holocene (for example, insolation-driven strongly enhanced Nile run-off during the intense wet phase of the NP after 12 kyr ago [11] , [12] (Nile experiment), the onset of Black Sea outflow [17] , [18] , [19] , enhanced northern borderland precipitation [14] , and enhanced run-off fed by meltwater from nearby mountainous glaciers [16] ). Their combined effect should have lifted the VSI and enhanced the deep-water oxygen consumption and together they determined the vertical extent and duration of S1 anoxia. In summary, we provide model and proxy data showing that the evolution of S1 anoxia occurred at the end of a long phase of deep-water stagnation, which was essentially preconditioned during or near the end of H1. Significantly, strongly and permanently enhanced biological production is not a prerequisite for the evolution of anoxia. The timing and duration of the stagnation prelude are in line with the proposed mechanisms for ORL1 deposition in the western Mediterranean [5] , [34] . Our results yield a conceptual understanding on the influence of short-term climate fluctuations (for example, YD and NP) on the variability of the VSI and oxygen consumption. To further detangle the importance of individual climatic events and sea-level fluctuations on deep-water stagnation and oxygen consumption, transient model experiments of the deglaciation EMS are required, for which our results provide a mechanistic understanding. A similar late glacial preconditioning of the deep-water circulation may have also led or contributed to the formation of other late Quaternary sapropels deposited near major glacial terminations, such as S5, S9 and S10 ( Supplementary Fig. 13 , Supplementary Note 5 ). Since at least sapropel S1, and possibly also S5, S9 and S10 are the result of a complex interplay between regional and large-scale climatic patterns (for example, warming, sea-level rise, insolation-driven enhanced African run-off) and ocean-biogeochemical mechanisms (for example, enhanced late glacial nutrient content and/or major shifts in the pelagic ecosystem structure) sapropel formation in general cannot be attributed to a single climatic event as was commonly proposed with the Nile hypothesis. Model description We use the Max Planck Institute ocean model (MPIOM) [56] coupled to the Hamburg ocean carbon cycle model (HAMOCC5) [57] , [58] , [59] . These models are developed by and available from the Max Planck Institute for Meteorology. The model domain used in this study covers the entire Mediterranean Sea and a small part of the Atlantic Ocean [33] , [47] , with a horizontal resolution of around 20 km, and 46 levels in the vertical. To account for the ∼ 20-m sea-level reduction during the early Holocene (relative to today), we reduce the depth of each grid box by adding the anomalies between the present-day and the early Holocene topography (derived from the ICE-5G reconstructions [60] ) to the standard topography. Consequently, the model sill depth of the Strait of Gibraltar is reduced from 256 to 241 m, and the Bosphorus is closed. The atmospheric forcing is derived from global climate model experiments of the 9 kyr ago Holocene insolation maximum (HIM) time slice, performed with the atmosphere-ocean-dynamical vegetation model (ECHAM5(T31,L19)/MPIOM(GR30,L40)/LPJ). We use a 100-year daily atmospheric data set to force the regional ocean-biogeochemical model in a repeating loop. A detailed description of the generation of the atmospheric forcing is given in Adloff et al . [47] . At the western boundary of the Atlantic Ocean box, a restoring to temperature, salinity, dissolved phosphate, dissolved nitrate, dissolved silica, dissolved oxygen and alkalinity is applied as detailed in Adloff et al . [47] and Grimm [59] . We added the differences of the river discharges (simulated by the global coupled climate model of the HIM time slice) to monthly climatological values of river run-off derived from the UNESCO RivDis database [61] . The river discharge, as well as dissolved phosphate and nitrate fluxes, is summarized in Supplementary Table 1 . See Grimm [59] for more details on how these nutrient fluxes were derived. The POC flux through the water column is divided into a slow sinking dead phytoplankton and zooplankton pool, and a fast sinking zooplankton fecal pellets pool [59] . Both POC classes are remineralized with a constant rate of 0.025 per day, and each class has its own sinking velocity set to constant values of 1.5 and 25 m per day. In the sediment, POC remineralization is dependent on bottom-water temperature [59] . POC is eroded using a physical erosion scheme, in which the strength of erosion is dependent on fluid motion [59] , [62] . Model spin-up and experimental design The model was initialized from homogeneous water conditions ( Supplementary Table 2 ). After an ocean-only spin-up experiment of 500 years, we coupled the physical ocean model to the biogeochemical model, which was also initialized with homogeneous water and sediment conditions ( Supplementary Table 2 ). The coupled ocean-biogeochemical model was run until the year 1,500. At the year 1,501, we increased the vertical resolution from 29 to 46 vertical layers, and integrated it for an additional 100 years. The entire 1,600 years of simulation served as a spin-up experiment. All model experiments examining the hypotheses 0 to 4 ( Table 1 ) for S1 formation were initialized from the spin-up experiment, with the perturbation scenarios chosen to approximate the very extreme end members of each hypothesis. We evaluate whether a particular hypothesis is plausible, and whether it is consistent with observational records. Criteria for plausibility are the time required to develop deep-water anoxia, the POC burial flux before and during S1 formation, and the vertical extent and duration of deep-water anoxia; all of these are readily compared with information derived from sediment records and proxy data. In the following, we describe the model experiments in more detail. Baseline experiment . In this experiment, we continued the spin-up experiment for another 4,100 years of simulation. The Baseline experiment serves as an early Holocene control experiment. 3xNutri experiment . Here we tripled the riverine nutrient input of all rivers draining into the Mediterranean Sea. To our knowledge, there are no quantitative reconstructions of riverine nutrient input data available for the early Holocene time slice. We assume that a tripled nutrient input describes an extreme upper range of the terrestrial nutrient input, although, our tripled riverine nutrient input to the EMS is considerably lower ( Supplementary Table 1 , 99.8 mol P s −1 ) than the high nutrient input experiment of a previous marine biogeochemical modelling study of S1 formation (125 mol P s −1 ) [21] . Nile experiment . Here we increased the Nile river run-off from 5,358 m 3 s −1 (used in the spin-up experiment) by adding another 9,000 m 3 s −1 . Compared with the estimated Nile discharge of ∼ 10,100 m 3 s −1 during the NP [63] , our Nile river discharge is even higher. Thus, our Nile experiment corresponds to a rather extreme permanent peak Nile run-off situation. In addition to the enhanced freshwater run-off, more nutrients are transported with the Nile river. We implement the default nutrient load to be proportional to the river freshwater run-off. Consequently, the Nile river in this experiment has a larger nutrient load than the Nile river in the Baseline experiment. This corresponds to nearly a doubling of the default total phosphate load (Baseline experiment) of all rivers draining into the EMS in the Nile experiment. The EMS nutrient input rate in the Nile experiment ( Supplementary Table 1 , 61.7 mol P s −1 ) is comparable to the rate of a low nutrient input experiment (65 mol P s −1 ) in a previous marine biogeochemical modelling study for S1 formation [21] . IniGlac experiment . The difference in the deep EMS water properties between the LGM and the Holocene corresponds to −3.1 °C for temperature and +2.1 p.s.u. for salinity [33] . With the IniGlac experiment we want to approximate the late glacial state sometime around H1. Therefore, we impose onto the last time step of the spin-up experiment the anomaly of the deep-water properties formed during H1 and force it with the HIM boundary conditions. Since H1 is a rather cold climate event [64] , we initialized the temperature change to be rather similar to the LGM state by imposing −3 °C onto the physical ocean state. In contrast, for salinity we impose only +1.5 p.s.u., since we assume that the increasing exchange rate at the Strait of Gibraltar has already led to a considerable freshening of the Mediterranean Sea since the LGM. Biogeochemical quantities were not modified. IniGlac+3xNutri experiment . Here we simulate the combination of a stagnating deep-water circulation (induced by climatic changes associated with the last late glacial to interglacial transition: IniGlac experiment) and enhanced biological production (stimulated by tripled nutrient inputs from rivers: 3xNutri experiment). In all experiments, the initial conditions of the biogeochemical traces in the water column were taken from the last time step of the spin-up experiment, and thus represent early Holocene nutrient-poor conditions. For the IniGlac and IniGlac+3xNutri experiment, these early Holocene highly oligotrophic and well-oxygenated conditions are inconsistent with the late glacial physical state. However, to our knowledge, there are no estimates for late glacial nutrient and oxygen conditions available. Apparent water age To assess the strength of mixing and stagnation, we introduce the apparent water age tracer ( A M ) in the model. This tracer increases its value linearly with time t in all locations i, j , and in all depth levels z , except for the surface, z surface , where it is kept at 0: Water age deviation The water age deviation ( A D ) is the fraction of the deviation of the simulated water age from the perfect stagnation (linear water aging, every year the water gets one year older), calculated as: where A T is the theoretical age the water would have under a perfect stagnation. We started this computation after 300 years of simulation to avoid the imprint of initialization effects. Negative values indicate that A M is older than the actual time elapsed, resulting from advection and/or mixing of older water from intermediate layers into greater depths. Positive values indicate the deviation from the perfect stagnation. Contrary to oxygen, the definition of A D is free of any imprint of biological processes, and thus shows the strength of mixing and stagnation. Ventilation–stagnation interface By assuming that A D >30% indicates well to intermittent ventilation, and lower values indicate stagnant conditions, we use A D =30% as a measure for the depth of the VSI. We choose this diagnostic to fit with the evolution of the oxygen profiles of all stagnation experiments. Proxy data and age models The age models for the evaluated proxy records are based on a combination of tephrochronology and radiocarbon dating of the test carbonate of surface-dwelling planktonic foraminifera [7] , [16] , [23] , [54] . AMS 14 C ages of sediment cores SL71, SL112, SL123 and SL148 have been transferred to calendar years by applying the Fairbanks 0805 calendar age conversion software [65] and considering an average EMS marine reservoir age of 400 years [66] . AMS 14 C ages of sediment cores LC-21, LC-31, SLA-9 and SL78 have been transferred to calendar years by applying the marine mode of the online version of CALIB 5.01 and considering a marine reservoir age of 420 years [67] . On the basis of the AMS 14 C analytical errors, different calibration software used, and consideration of different reservoir ages, dating uncertainties range from ∼ ±250 years during the Late glacial to ±50 years during the late Holocene period [7] . Stable isotope measurements Planktonic and benthic foraminiferal stable isotope data have been compiled from literature sources and unpublished data. The methodology follows that described in previous studies [51] , [54] , [68] , [69] . For the present study, at least 10 tests of the planktonic foraminifera Globigerinoides ruber (white) were picked from the >150-μm fraction for δ 13 C measurements. Benthic epifaunal taxa such as Cibicidoides spp. and Planulina ariminensis have been selected for δ 13 C measurements at upper bathyal sites. At lower bathyal and abyssal sites, alternative (preferentially epifaunal rotaliid and miliolid species) had to be considered due to a lack of the aforementioned taxa. Paired measurements of miliolid and rotaliid species suggest a δ 13 C vital effect of larger than +1% for Miliolinella subrotunda . Depending on species-specific test sizes and availability, up to 10 benthic foraminiferal tests were selected from the >125 or >150-μm size fractions. Stable isotope measurements were carried out at different intercalibrated mass spectrometer facilities with an external precision better than 0.03–0.06% for stable carbon isotopes [7] , [37] , [54] , [68] , [69] . How to cite this article: Grimm, R. et al . Late glacial initiation of Holocene eastern Mediterranean sapropel formation. Nat. Commun . 6:7099 doi: 10.1038/ncomms8099 (2015).